Palladium-catalyzed allene synthesis enabled byβ-hydrogen elimination fromsp2-carbon The rational design based on a deep understanding of the present reaction mechanism is an important, viable approach to discover new organic transformations. β -Hydrogen elimination from palladium complexes is a fundamental reaction in palladium catalysis. Normally, the eliminated β- hydrogen has to be attached to a sp 3 -carbon. We envision that the hydrogen elimination from sp 2 -carbon is possible by using thoroughly designed reaction systems, which may offer a new strategy for the preparation of allenes. Here, we describe a palladium-catalyzed cross-coupling of 2,2-diarylvinyl bromides and diazo compounds, where a β -vinylic hydrogen elimination from allylic palladium intermediate is proposed to be the key step. Both aryl diazo carbonyl compounds and N -tosylhydrazones are competent carbene precursors in this reaction. The reaction mechanism is explored by control experiments, KIE studies and DFT calculations. Palladium catalysis has proved to be a powerful synthetic tool, which is demonstrated by numerous useful transformations and highlighted by the 2010 Nobel Prize in chemistry [1] , [2] , [3] . Although the mechanism involved in those reactions have been extensively explored, efforts to acquire a deep understanding of the current mechanistic hypothesis and apply them to design new transformations have never ceased. As an elementary reaction in palladium catalysis, β -hydrogen elimination has been well studied (Fig. 1a ) [4] , [5] , [6] , [7] . Theoretically, the hydrogen elimination can be divided into two categories according to the hybrid state of the attached carbon atom. Hydrogen elimination from sp 3 -carbon is the most common pattern, and both alkyl and alkenyl palladium complexes [8] , [9] , [10] , [11] can undergo this elimination pathway, affording olefins and allenes respectively. In contrast, the second hydrogen mode, where the eliminated hydrogen is attached to a sp 2 -carbon (also means β -elimination of vinylic hydrogen from 1 η - δ -allylic palladium) and allene would be generated, has not been reported yet (Fig. 1b ). Fig. 1: Allene synthesis based on β -hydrogen elimination from sp 2 hybrid carbon. a β -Hydrogen elimination in palladium catalysis. b Two modes of β -hydrogen elimination. c Allene synthesis via β -hydrogen elimination from C( sp 2 ) (this work). Full size image On the other hand, allenes are of great importance due to their wide existence in natural products [12] , pharmaceuticals [13] , and molecular materials [14] . The active nature imparted by its unique orthogonal cumulative π -system also makes them highly versatile and useful building blocks in organic synthesis [15] , [16] , [17] , [18] , [19] . Although numerous methods for the preparation of allenes have been developed [20] , [21] , [22] , [23] , [24] , they still lag far behind the growing demand in the application. At present, the majority of the existing methodologies rely on the utilization of elaborate alkynes. Therefore, it is highly desirable to develop new approaches via new mechanistic pathways, which may deliver the allenes efficiently from easily accessible starting materials and complement the current methodologies [25] , [26] , [27] , [28] , [29] , [30] , [31] , [32] , [33] . Therefore, β -hydrogen elimination of allylic palladium from sp 2 -carbon represents an attractive new strategy for allene synthesis. Here, we report the successful application of the β -hydrogen elimination from sp 2 -carbon for the allene synthesis. In our research plan, the desired δ -allylic palladium intermediate is planned to be produced from the classic allylic alcohol derivatives, which can undergo an oxidative addition/isomerization sequence in the presence of Pd 0 (Fig. 1c , pathway I). A second pathway was also devised where the cross-coupling of alkenyl halides and diazo compounds offer the desired δ -allylic palladium intermediate via migratory of palladium carbene IV (Fig. 1c , pathway II) [34] , [35] , [36] , [37] . In these two pathways, there is an equilibrium of 1 η - δ - and 3 η-π -allylic palladium intermediates. The π -allylic palladium normally showed higher stability compared with the corresponding δ -allylic one. However, The lack of a syn coplanar arrangement of C–H and C-Pd bonds, a key factor for most β -hydrogen elimination, would make the hydrogen elimination from π -allylic palladium rather difficult [38] , [39] , [40] . Initial study With these considerations in mind, we set out to explore the feasibility of the planned strategy. A small amount of allene 2 was observed when allyl acetate 1 was treated by Pd(OAc) 2 /PPh 3 at 100 o C with poor conversion (Fig. 2a ). However, attempts to further improve this reaction were unsuccessful, and a complicated mixture was observed when a full conversion was achieved by changing ligands or solvents. Next, we tested the cross-coupling of 2,2-diarylvinyl bromide 3a and diazoacetate 4a in the presence of Pd(OAc) 2 /PPh 3 (Fig. 2b ). These two model substrates were selected because the planned elimination is expected to be promoted by the generation of stable multi-aryl substituted allenes, and the competitive elimination from a sp 3 -carbon will be avoided. Delightfully, the desired allene 5a was generated in high yield, and its structure was unambiguously confirmed by X-ray analysis. Fig. 2: Initial studies. a Allene synthesis starting from allyl acetate 1 . b Allene synthesis starting from vinylbromide 3a and diazoacetate 4a . 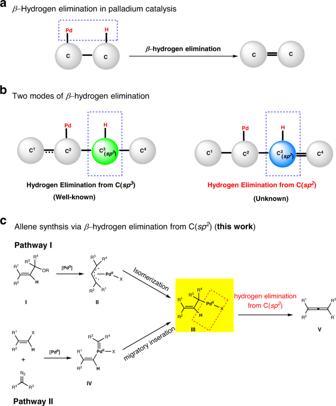Fig. 1: Allene synthesis based onβ-hydrogen elimination fromsp2hybrid carbon. aβ-Hydrogen elimination in palladium catalysis.bTwo modes ofβ-hydrogen elimination.cAllene synthesis viaβ-hydrogen elimination from C(sp2) (this work). Full size image Reaction conditions development Encouraged by the above results, more reaction conditions were screened for a higher reaction yield (Table 1 ). Other mono-phosphine ligands, with either electron-withdrawing fluorine (L2) or electron-donating MeO group (L3), gave reduced reaction yields (entries 2 and 3). Bis-phosphine ligands were also competent to promote this reaction, and the ligand bearing a linkage of six carbon atoms further improved the reaction yield to 87% (entries 4–7). Instead of CsOAc, several other bases were also examined, but offered inferior results (entries 8–10). The reaction also went well in other ether solvents, but was rather sluggish with toluene or DCE as solvent (entries 13 and 14). While a comparable result was obtained in an elevated reaction temperature of 90 o C (entry 15), an obvious loss in reaction yield was observed at a lower temperature (entries 16 and 17). Table 1 Optimization of reaction conditions. Full size table Substrate scope of 2,2-diarylvinyl bromides with diazo carbonyl compounds With the optimal reaction conditions in hand, we began to explore the generality of this cross-coupling reaction (Fig. 3 ). First, a variety of 2,2-diarylvinyl bromides 3 were used in the coupling with phenyl diazoacetate 4a . All of them afforded high yields, with a deleterious effect on the reaction outcome by introducing electron-withdrawing groups to the phenyl ring, or moving the substituents from para - to meta- or ortho- position ( 5d–i ). Vinyl bromide with a flat terminal fluorene substitution, instead of two separate aryl groups, also proceeded well ( 5l ). Next, the variation of the aryl diazoacetates 4 was also investigated. The methyl ester could be successfully replaced by an ethyl or benzyl ester, as well as an ethyl ketone ( 5m–o ). Introduction of different substituents onto the para- or meta- position of the phenyl ring was well tolerated, albeit in slightly reduced reaction yields ( 5p–w ). Compared with the vinyl bromide substrates, the diazoacetate part was more sensitive to the steric properties, as the ortho- methyl substituted phenyl ring completely blocked the coupling reaction ( 5x ). Delightfully, other aromatic rings, like 2-thienyl or naphthyl group, could provide the desired products in good yields ( 5y and 5z ). Fig. 3: Cross-coupling of 2,2-diarylvinyl bromides with diazo carbonyl compounds. a Reactions conditions: 3 (0.20 mmol), 4 (0.30 mmol, 1.5 equiv), Pd(OAc) 2 (0.02 mmol, 0.1 equiv), dpph (0.03 mmol, 0.15 equiv), CsOAc (0.30 mmol, 1.5 equiv), THF (2 mL), 80 o C. Isolated yields. Full size image Substrate scope of 2,2-diarylvinyl bromides with N -tosylhydrazones Encouraged by the above success, we sought to use diaryldiazomethanes to produce tetra-aryl-substituted allenes, which showed some unique properties in material science [41] , catalysis [42] , [43] , and molecular recognition [44] , [45] . Although a preliminary experiment with diphenyldiazomethane furnished the tetra-phenyl-substituted allene 7a in moderate reaction yield under the standard reaction conditions, further efforts were hampered by the relatively lower stability of this kind of diazo compounds. Therefore, we switched to the corresponding N -tosylhydrazones 6 , a family of stable carbene precursors [46] , [47] , [48] . Gratifyingly, the slight adjustment of the base and ligand to cesium pivalate and dppe could lead to the desired cross-coupling products in good to excellent yields (Fig. 4 ). While electronic variation on the phenyl ring of the 2,2-diarylvinyl bromides showed marginal effect on the reaction outcome ( 7a–h ), the introduction of electron-withdrawing groups to the diaryl ketones derived N -tosylhydrazones gave slightly reduced yields ( 7j–l ). Ortho -substituted phenyl rings on either vinyl bromides or N -tosylhydrazone part resulted in an obvious loss in reaction yield, consistent with results from diazoacetate species ( 7g and 7n ). Fig. 4: Cross-coupling of 2,2-diarylvinyl bromides with N -tosylhydrazones. a Reaction conditions: 3 (0.20 mmol), 6 (0.30 mmol, 1.5 equiv. ), Pd(OAc) 2 (0.02 mmol, 0.1 equiv. ), dppe (0.03 mmol, 0.15 equiv. ), CsOPiv (1.00 mmol, 5 equiv. ), THF (5 mL), 80 o C. Isolated yields. Full size image Conversion of the obtained product The conversion of allene 5a was tested (Fig. 5 ). In the presence of a rhodium catalyst, the allenic esters can be selectively borylated by B 2 (pin) 2 to afford vinyl boronate pinacol ester 8a in 78% yield. According to the previous report [49] , the allenic esters can also undergo a sequential nucleophilic attack/cyclization process to give polysubstituted α-naphthol 8b in moderate yield. Treatment of 5a with TfOH afforded allenic carboxylic acid 8c in 78% yield, which may be used to attach this unique allene architecture to other molecules. Fig. 5: Conversion of the obtained product 5a. Reaction conditions and isolated yield are reported along the arrows. Full size image Control experiments To probe the mechanism of this catalytic reaction, palladium complex 9 was prepared and subjected to several control experiments (Fig. 6 ). Palladium complex 9 was prepared by reaction of 2,2-diphenylvinyl bromide 3a and Pd(PPh 3 ) 4 , and the structure was verified by X-ray crystallographic analysis. See SI for details. Fig. 6: Control experiments with palladium complex. a Reaction of palladium complex 9 and diazoacetate 4a at 80 o C in the absence of base. b Reaction of palladium complex 9 and diazoacetate 4a at 110 o C in the absence of base. c Reaction of palladium complex 9 and diazoacetate 4a at 80 o C in the presence of CsOAc. Full size image When the mixture of complex 9 and diazoacetate 4a in THF was heated at 80 o C for 2 h, the reaction solely afforded olefin 10 (Fig. 6a ). The reaction mixture was also analyzed by SAESI-HRMS, which is a direct and reliable method for the characterization of reaction intermediates in situ through a gentle ionization process [50] , [51] , [52] , [53] . The obtained MS spectrum showed a signal of palladium complex [C 59 H 49 O 2 P 2 Pd] + . The peaks in MS spectrum labeled as experimental m/z -relative percentage abundance matched the theoretical shown in brackets, unambiguously indicating the existence of allylic palladium species 11 . The relative abundance of the isotopic ion at m/z 959.2242 was higher than the theoretical value due to the influence of the background signal nearby. A small amount of allene 5a could be observed upon elevation of reaction temperature, with olefin 10 still as the major product (Fig. 6b ). However, the preference of reaction products was completely inverted when cesium acetate was added, and only allene 5a was produced even at 80 o C (Fig. 6c ). These experiments hint that the reaction generated an allylpalladium intermediate, which could undergo either protodepalladation [54] to afford olefin 10 , or hydrogen elimination to give allene 5a . Such a hydrogen elimination step can be facilitated by the basic carboxylate salts. KIE and deuterium-labeling experiments To gain more mechanistic insights, two deuterium labeling experiments were carried out (Fig. 7 ). The kinetic isotope effect (KIE) was measured in two parallel reactions using 3a and deuterium-labeled d 1 -3a . A KIE value of 1.02 implicated that the final hydrogen elimination was not involved in the rate-limiting step [55] . In the presence of 4 equivalents of D 2 O, the reaction of complex 9 and diazoacetate 4a afforded deuterated olefin d 1 - 10 with 71% D incorporation, showing the possibility of the protodepalladation by the moisture of the reaction system in the absence of a carboxylate salt. Fig. 7: KIE and deuterium-labeling experiments. a KIE determined from two parallel reactions. b Deuterium incorporation experiment. Full size image Proposed reaction mechanism Based on the above investigations and literature precedents, a plausible mechanism is outlined in Fig. 8 . Initially, oxidative addition of vinyl bromide 3a to the Pd 0 catalyst offers the Pd II species A . Then the Pd II species A reacts with the diazoacetate 4a to form Pd II carbene species B . A subsequent migratory insertion of carbene into the Pd−C bond affords π -allylpalladium species C [56] , [57] , [58] , [59] , which is followed by a hydrogen-elimination to provide the desired product 5a . Fig. 8: Plausible reaction mechanism. X = Br or OAc; ligands are omitted for clarity. Full size image DFT calculations To gain a deeper understanding of the palladium-catalyzed cross-coupling of vinyl bromides with diazo compounds, DFT calculations were carried out for the envisioned reaction intermediates and related transition states (Fig. 9 , see computational details in the Supplementary Information ). Fig. 9: Energy profiles and geometries of key species for the tentative reaction pathways. a Energy profiles and geometries of key species for the formation of allylpalladium species. b Energy profiles and geometries of key species for β -hydrogen elimination mechanism. All results are calculated at the SMD (tetrahydrofuran) M06/def2-TZVP//B3LYP/6-31G(d)(LANL2DZ) level of theory. Relative free energies are in kcal/mol and bond lengths are in Å. Full size image As can be seen from Fig. 9a , the oxidative addition of vinylbromide 3a to the Pd(0)L 2 complex (L = PPh 3 ), which is exergonic by 9.1 kcal/mol with an energy barrier of 12.7 kcal/mol, initiates the reaction and offers bromide coordinated species Int2 . Isomerization of Int2 by exchanging the positions of vinyl ligand and PPh 3 ligand forms a more stable isomer Int3 . We also explored the reaction pathway initiated by the addition of diazo compound with Pd(0)L 2 . However, as the dediazonation process in this pathway requires a high free energy barrier of 33.2 kcal/mol (see Supplementary Fig. 4 in Supplementary Information), such a mechanism will not be further considered. The subsequent addition of diazoacetate 4a to Int3 with simultaneous dissociation of one PPh 3 group is endergonic by 22.3 kcal/mol and leads to Int4 in which diazoacetate weakly occupies the vacant site of Pd(II). Further reaction of diazoacetate with Pd(II) center releases a molecule of nitrogen and leads to a Pd(II) carbene intermediate Int5 . This step is calculated to be 18.8 kcal/mol exothermic with an energy barrier of 9.8 kcal/mol. A subsequent migratory insertion of the generated carbene into the Pd−C bond of Int5 affording the π -allylpalladium species Int6 is further exothermic by 47.7 kcal/mol without any energy barrier. We also investigated an alternative reaction pathway for π -allylpalladium species formation, in which ligand exchange of bromide with the base CsOAc happens before dediazonation and migratory insertion (see Supplementary Fig. 2 in Supplementary Information). However, with an overall energy barrier of about 36.4 kcal/mol, this reaction pathway seems to be unfavorable in practice and thus will not be discussed further. Nevertheless, as shown in Fig. 9b , the ligand exchange indeed takes place after the formation of Int6 to produce base coordinated π -allylpalladium species Int7 with an endergonic reaction energy of 3.2 kcal/mol. The so-generated Int7 then undergoes β -hydrogen elimination to provide the desired allene product. At this stage, two alternative pathways, of which one involves the coordinated base (path A in Fig. 9b ) while the other involves the palladium center (path B in Fig. 9b ), were investigated respectively. As depicted in path A, isomerization of Int7 to δ-palladium tetra -coordinated intermediate Int8 is endergonic by 11.2 kcal/mol, with the base AcO − acting as a bidentate chelate ligand and β -hydrogen of allyl ligand getting close to one of the oxygen atoms of AcO − . The resulting Int8 then undergoes base promoted β -hydrogen elimination through a bicyclo[4.1.0] transition state ( TS4 ) to afford allene coordinated complex ( Int9 ) with a small energy barrier of 7.8 kcal/mol accompanying with an exothermicity of 6.1 kcal/mol. Finally, the Pd(0)L 2 coordinated with allene is restored by ligand exchange between the coordinated AcOH of Int9 and PPh 3 with an exergonic reaction energy of 12.6 kcal/mol indicating that the whole reaction is thermodynamically favorable. In contrast, due to the sterically more crowded structure possessed in the isomer Int10 and the larger tension of the four-membered ring transition state ( TS5 ), the reaction mechanism via path B is energetically unfavorable. As such, the results from our DFT calculations suggest that palladium-catalyzed cross-coupling of 2,2-diarylvinylbromides with diazo compounds to produce allenes involves base promoted β -hydrogen elimination mechanism. The rate-determining step is found to be dediazonation with the overall energy barrier of 32.1 kcal/mol ( TS2 vs Int3 in Fig. 9a ), which is somewhat high considering the reaction temperature of 80 o C, possibly due to the insufficient accuracy of DFT methods in some cases. The experimentally observed small KIE supports the DFT results that β -hydrogen elimination is not the rate-determining step (for computational details, see Supplementary Data 1 ). In summary, We have developed a highly efficient palladium-catalyzed cross-coupling of 2,2-diarylvinyl bromides with diazo compounds for the modular synthesis of tetrasubstituted allenes. The reaction can be promoted by either mono - or bis-phosphine ligands, and ligand dpph with a flexible six-carbon linkage proved to be the optimal choice. Under optimized conditions, both aryl diazoacetates and N -tosylhydrazones are competent coupling partners. To gain insight into the reaction mechanism, control experiments, KIE studies, and DFT calculations were carried out. The key step in the catalytic cycle is believed to undergo a β -vinylic hydrogen elimination from allyl palladium intermediate, where acetate anion acts as an inner base to form a bicyclo[4.1.0] transition state. The computational study also indicates that the rate-determining step is dediazonation with the overall energy barrier of 32.1 kcal/mol. Notably, the β -hydrogen elimination mode revealed by the present work deepened our understanding of this elementary step in palladium catalysis and paved a new way for the allene synthesis. 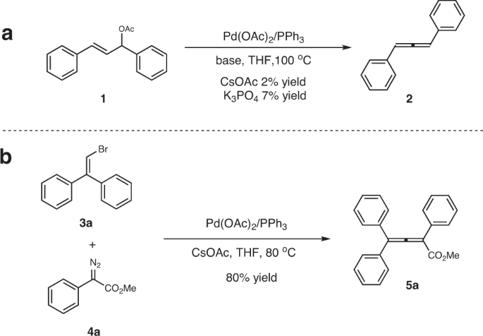Fig. 2: Initial studies. aAllene synthesis starting from allyl acetate1.bAllene synthesis starting from vinylbromide3aand diazoacetate4a. Typical procedure for coupling of 2,2-diarylvinyl bromides with diazo carbonyl compounds To a 25 mL Schlenk tube charged with a stir bar, 2,2-diarylvinyl bromides ( 3 ) (0.2 mmol), α-diazoesters ( 4 ) (0.3 mmol), Pd(OAc) 2 (4.48 mg, 0.02 mmol), dpph (13.6 mg, 0.03 mmol) and CsOAc (58 mg, 0.3 mmol) were added. After filled with argon, anhydrous THF (2 mL) were added via a syringe. The mixture was stirred at 80 °C in an oil bath for 2 h. Upon completion, the reaction mixture was washed with brine (15 mL) and extracted with EtOAc (3 × 10 mL). The combined organic phases were dried over anhydrous Na 2 SO 4 , filtered, and concentrated under reduced pressure. The crude products were purified by silica gel chromatography (petroleum ether/EtOAc = 20:1 ~ 5:1) to afford pure products ( 5 ). Typical procedure for 2,2-diarylvinyl bromides with N -tosylhydrazones To a 25 mL Schlenk tube charged with a stir bar, 2,2-diarylvinyl bromides ( 3 ) (0.2 mmol), N -tosylhydrazones ( 6 ) (0.3 mmol), Pd(OAc) 2 (4.48 mg, 0.02 mmol), DPPE (11.9 mg, 0.03 mmol) and CsOPiv (234 mg, 1 mmol) were added. After filled with argon, anhydrous THF (5 mL) was added via a syringe. The mixture was stirred at 80 °C in an oil bath for 4 h. Upon completion, the reaction mixture was washed with brine (15 mL) and extracted with EtOAc (3 × 10 mL). The combined organic phases were dried over anhydrous Na 2 SO 4 , filtered, and concentrated under reduced pressure. 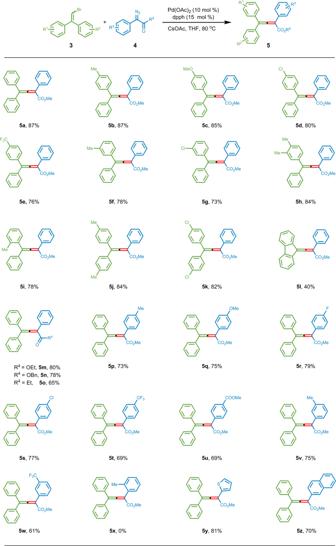Fig. 3: Cross-coupling of 2,2-diarylvinyl bromides with diazo carbonyl compounds. aReactions conditions:3(0.20 mmol),4(0.30 mmol, 1.5 equiv), Pd(OAc)2(0.02 mmol, 0.1 equiv), dpph (0.03 mmol, 0.15 equiv), CsOAc (0.30 mmol, 1.5 equiv), THF (2 mL), 80oC. Isolated yields. 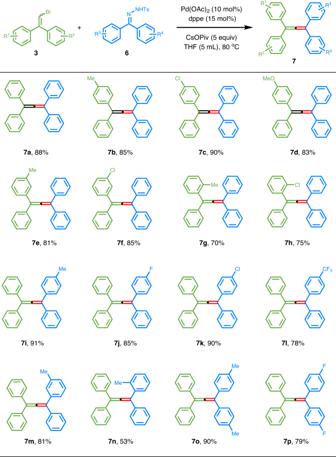Fig. 4: Cross-coupling of 2,2-diarylvinyl bromides withN-tosylhydrazones. aReaction conditions:3(0.20 mmol),6(0.30 mmol, 1.5 equiv.), Pd(OAc)2(0.02 mmol, 0.1 equiv.), dppe (0.03 mmol, 0.15 equiv.), CsOPiv (1.00 mmol, 5 equiv.), THF (5 mL), 80oC. Isolated yields. 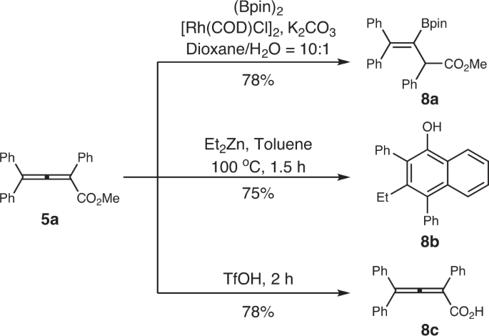Fig. 5: Conversion of the obtained product 5a. Reaction conditions and isolated yield are reported along the arrows. 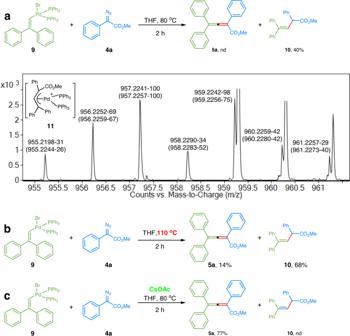Fig. 6: Control experiments with palladium complex. aReaction of palladium complex9and diazoacetate4aat 80oC in the absence of base.bReaction of palladium complex9and diazoacetate4aat 110oC in the absence of base.cReaction of palladium complex9and diazoacetate4aat 80oC in the presence of CsOAc. 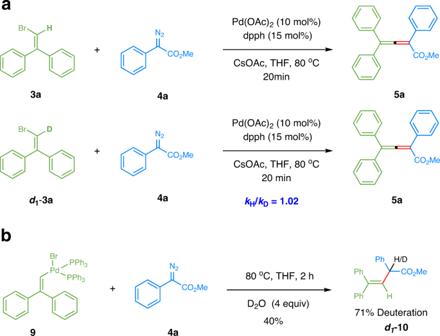Fig. 7: KIE and deuterium-labeling experiments. aKIE determined from two parallel reactions.bDeuterium incorporation experiment. 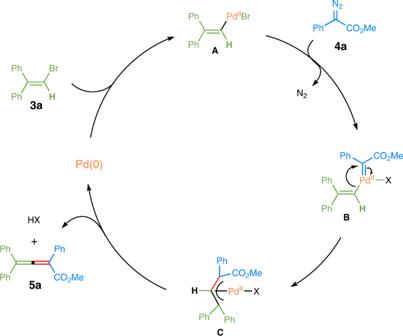Fig. 8: Plausible reaction mechanism. X = Br or OAc; ligands are omitted for clarity. 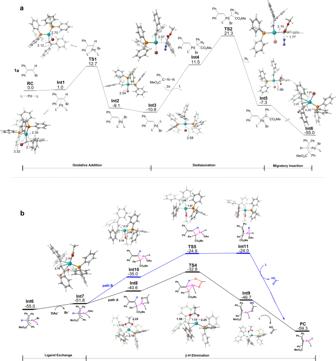Fig. 9: Energy profiles and geometries of key species for the tentative reaction pathways. aEnergy profiles and geometries of key species for the formation of allylpalladium species.bEnergy profiles and geometries of key species forβ-hydrogen elimination mechanism. All results are calculated at the SMD (tetrahydrofuran) M06/def2-TZVP//B3LYP/6-31G(d)(LANL2DZ) level of theory. Relative free energies are in kcal/mol and bond lengths are in Å. The crude products were purified by silica gel chromatography (petroleum ether/EtOAc = 100:1 ~ 20:1) to afford pure products ( 7 ).